Spin-enhanced organic bulk heterojunction photovoltaic solar cells Recently, much effort has been devoted to improve the efficiency of organic photovoltaic solar cells based on blends of donors and acceptors molecules in bulk heterojunction architecture. One of the major losses in organic photovoltaic devices has been recombination of polaron pairs at the donor–acceptor domain interfaces. Here, we present a novel method to suppress polaron pair recombination at the donor–acceptor domain interfaces and thus improve the organic photovoltaic solar cell efficiency, by doping the device active layer with spin 1/2 radical galvinoxyl. At an optimal doping level of 3 wt%, the efficiency of a standard poly(3-hexylthiophene)/1-(3-(methoxycarbonyl)propyl)-1-1-phenyl)(6,6)C 61 solar cell improves by 18%. A spin-flip mechanism is proposed and supported by magneto-photocurrent measurements, as well as by density functional theory calculations in which polaron pair recombination rate is suppressed by resonant exchange interaction between the spin 1/2 radicals and charged acceptors, which convert the polaron pair spin state from singlet to triplet. Solar energy has been identified as the leading renewable energy source to meet the challenge of increasing energy demand. Organic photovoltaics [1] , [2] , [3] , [4] , [5] , [6] , [7] , [8] , [9] , [10] , [11] , [12] , [13] , [14] , [15] , [16] , [17] , [18] , [19] , [20] , [21] , [22] , [23] , [24] , [25] (OPV) represent an emerging sector in the photovoltaic industry that has seen a rapid development in recent years. Compared to the 3% power conversion efficiency ( η ) value reported in 2007 (ref. 26 ), to date the best OPV solar cell that employs a non-tandem bulk heterojunction (BHJ) structure has shown η ~8.3% [27] . In a typical BHJ architecture (see Fig. 1a for a typical OPV device), a solvent-cast layer of π-conjugated polymer and fullerene-derivative blend is sandwiched between the cathode and anode. The most studied polymer/fullerene blend with high η -value comprises of regio-regular poly(3-hexylthiophene) (P3HT) (donor—D) and 1-(3-(methoxycarbonyl)propyl)-1-1-phenyl)(6,6)C 61 (PCBM) (acceptor—A), of which chemical structures are shown in Fig. 1a . This blend is known to contain separate D and A nano-sized domains that facilitate both charge photogeneration and charge transport, and collection in the blend [3] , [4] . The P3HT donor polymer absorbs in the UV-visible part of the solar spectrum that compensates the optical transparency of the fullerene molecules in the same energy range. Upon light absorption in the P3HT polymer chains, excitons are initially photogenerated in the donor nano-domains [28] ; their subsequent dissociation at the D–A interfaces is facilitated by the energy level difference between the lowest unoccupied molecular orbital (LUMO) of the donor and acceptor, as well as between their highest occupied molecular orbital (HOMO) levels. To reach the D–A interfaces, the excitons first diffuse towards the polymer domain boundary within ~10 ps [28] , [29] where upon arrival they form charge transfer excitons [30] , [31] . Subsequently, the charge-transfer excitons separate into Coulombically bound polaron pairs (PP), which are the intermediate species at the D–A domain interfaces having relatively long lifetime (namely, few microseconds) [32] . At a later time, the PP species may separate into 'free' electron and hole polarons available for charge transport via the A and D domains, and can be readily collected at the anode and cathode, respectively. 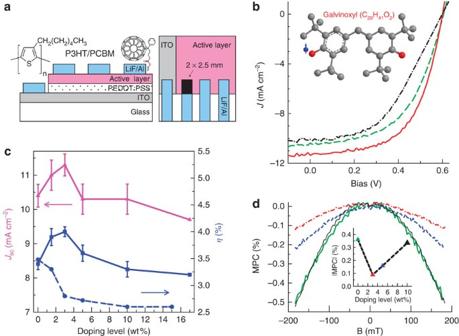Figure 1: Spin enhancement of OPV solar cell based on P3HT/PCBM blend doped with spin 1/2 galvinoxyl radicals. (a) The OPV cell structure (for fabrication see Methods). The P3HT repeat unit and PCBM molecular structure are also shown in the insets. (b) The I-V characteristics of OPV solar cells of pristine P3HT/PCBM blend (η=3.4%, dashed line), the blend doped with 3 wt% galvinoxyl radicals (η=4.0%, solid line) and the blend doped with 3 wt% precursor (η=2.8%, dash–dot line) under AM1.5 'sun illumination' condition. The inset shows the galvinoxyl molecular structure. Small sphere bisected by arrow denotes unpaired electron. (c) The change in OPV device properties with galvinoxyl-additive concentration,Jsc(triangles) andη(squares), are shown versus galvinoxyl wt% in the P3HT/PCBM blend.ηof OPV devices doped with galvinoxyl precursor that does not possess spin 1/2 radical is also shown for comparison (circles). (d) MPC response of OPV devices doped with galvinoxyl (pristine: thick-solid line; 3 wt%: dash–dot line; 5 wt%: dashed line; 10 wt%: thin-solid line) up to field,Bof 190 mT. The inset summarizes the MPC value at 150 mT versus galvinoxyl wt%. Figure 1: Spin enhancement of OPV solar cell based on P3HT/PCBM blend doped with spin 1/2 galvinoxyl radicals. ( a ) The OPV cell structure (for fabrication see Methods). The P3HT repeat unit and PCBM molecular structure are also shown in the insets. ( b ) The I-V characteristics of OPV solar cells of pristine P3HT/PCBM blend ( η =3.4%, dashed line), the blend doped with 3 wt% galvinoxyl radicals ( η =4.0%, solid line) and the blend doped with 3 wt% precursor ( η =2.8%, dash–dot line) under AM1.5 'sun illumination' condition. The inset shows the galvinoxyl molecular structure. Small sphere bisected by arrow denotes unpaired electron. ( c ) The change in OPV device properties with galvinoxyl-additive concentration, J sc (triangles) and η (squares), are shown versus galvinoxyl wt% in the P3HT/PCBM blend. η of OPV devices doped with galvinoxyl precursor that does not possess spin 1/2 radical is also shown for comparison (circles). ( d ) MPC response of OPV devices doped with galvinoxyl (pristine: thick-solid line; 3 wt%: dash–dot line; 5 wt%: dashed line; 10 wt%: thin-solid line) up to field, B of 190 mT. The inset summarizes the MPC value at 150 mT versus galvinoxyl wt%. Full size image One of the main challenges that OPV faces at the present time is its low η -value compared with other photovoltaic devices [1] , with the recombination of PP at D–A interfaces being a major limiting factor [29] , [33] , [34] , [35] . In addition to optimizing parameters such as material mass ratio, active layer thickness and annealing temperature, numerous other approaches have been tried to enhance the efficiency by improving the device morphology [2] , [3] , [4] , [5] , engineering new polymer/fullerene materials [6] , [7] , [8] , [9] , [10] , [11] , manipulating electrode property [12] , [13] , [14] , [15] , employing tandem cell architecture [16] , [17] , [18] and enhancing optical absorption [19] . A number of these approaches involve introducing nano-particles dopants (or additives) into the active layer and/or fabrication process [2] , [3] , [12] , [13] , [22] , [23] , [24] . In the present work, we demonstrate a new method to improve OPV efficiency by doping the device active layer with spin 1/2 radicals to reduce PP recombination at the polymer/fullerene interfaces. We achieved a significant increase in η by up to ~340% (in acceptor-rich devices) relative to devices based on pristine blends. We demonstrate that the spin 1/2 radical additives facilitate the intersystem crossing of PP from singlet to triplet spin configuration, thereby enhancing PP separation into free charges in the device; this process is unraveled via magneto-photocurrent (MPC) of the doped devices. We demonstrate that the spin 1/2 radicals may spin flip the acceptor electron spin via an exchange mechanism that requires resonant conditions. We believe that this method may work with other D–A blends if appropriate radicals in resonance are found, in concert with other existing methods to yield even higher OPV device efficiencies. Galvinoxyl-doped P3HT/PCBM OPV devices The spin 1/2 radical that enhances OPV performance in this work is galvinoxyl (2,6-di- t -butyl-α-(3,5-di- t -butyl-4-oxo-2,5-cyclohexadien-1-ylidene)- p -tolyloxy), a π-conjugated molecule with C 2 symmetry ( Fig. 1b inset). The bulky t -butyl groups on the molecule stabilize the radical by keeping other molecules apart thus preventing further radical–radical spin interaction in the solid state. The unpaired electron is delocalized over the entire molecule and thus its molecular structure may be regarded as resonance hybrid of two configurations having a localized unpaired spin-polarized electron on different oxygens [36] . First, we investigated the effect of galvinoxyl doping in the active layer of a 'standard' P3HT/PCBM device having 1.2:1 weight ratio. We note that our standard P3HT/PCBM devices were fabricated using a well-optimized recipe, and the obtained η -value is ~3.4%, which is close to the published value by Plextronics [37] ; it represents an upgrade from our preliminary results [38] . Figure 1b shows that by doping 3 wt% of galvinoxyl, η increases from 3.4 (short circuit current: J sc =10.4 mA cm −2 , open circuit voltage: V oc =0.6 V, fill factor: FF =0.56) to 4.0% ( J sc =11.3 mA cm −2 , V oc =0.6 V, FF =0.62) exhibiting an 18% enhancement in the power conversion efficiency. This η increase is significantly larger than the standard deviation in η -values of our optimal devices (±3%) ( Supplementary Table S1 ); thus, doping with galvinoxyl unambiguously enhances the device η -value. The 8.7% increase in J sc that accounts for about half of the improvement in the device η indicates that carrier photogeneration increases or carrier recombination is reduced, or both. Figure 1c summarizes the P3HT/PCBM (1.2:1) device properties for all investigated galvinoxyl concentrations (1.5–17 wt%). The enhancement in J sc and η induced by the galvinoxyl radicals peaks at ~3 wt% and gradually vanishes with further increased doping. Actually, at high doping level (>10 wt%) galvinoxyl suppresses the device performance. The optimal doping concentration (~3 wt%) at which η maximizes divides the effect of galvinoxyl additives into two regimes: an 'enhancement' regime, where η increases with doping, and a 'suppression' regime, where η decreases with doping. We also performed MPC measurements on the galvinoxyl-doped OPV devices to unravel the underlying mechanism for the increase in J sc with wt%. Figure 1d shows the obtained MPC response of OPV devices having various galvinoxyl wt%. It is clearly seen that galvinoxyl additives reduce the MPC value without changing the field response. It has been known that MPC in OPV blends is due to magnetic field manipulation of spin triplet and singlet states within the PP species [39] , [40] , [41] . Therefore, the reduction of MPC with wt% shows that the spin 1/2 radicals interfere with the intersystem crossing rates among the various spin states of the PP species, revealing the importance of the galvinoxyl spin rather than its ability to serve as donor or acceptor. We therefore conclude that reduced PP geminate recombination at the D–A interfaces is responsible for the enhanced carrier photogeneration upon galvinoxyl doping. The remaining enhancement in η with the galvinoxyl additives is due to an increase in FF , which indicates a reduced series resistance that results from improved carrier transport. We note that the MPC reduction with galvinoxyl wt% follows the same trend as that of the OPV enhancement with wt%. Figure 1d inset shows that the most MPC reduction occurs at 3 wt%; the MPC response comes back to that of pristine device at 10 wt%. This further shows the existing correlation between the spin 1/2 properties of the galvinoxyl additives and the OPV enhancement. In the following, we describe several 'control experiments' that we performed for understanding the OPV enhancement upon galvinoxyl doping. To investigate whether the enhancement in J sc with galvinoxyl doping is due to an increase in the device active layer absorption, we compared the absorption spectra of the pristine and galvinoxyl optimally doped P3HT/PCBM films ( Fig. 2a ). The two spectra are very similar to each other; and, in particular, the galvinoxyl absorption peak at 430 nm ( Fig. 2a ), which originates from HOMO–LUMO transition, is not discerned in the doped sample absorption. We therefore conclude that the enhancement in J sc is not caused by a change in absorption with galvinoxyl doping. In Fig. 2b, we compare the external quantum efficiency (EQE) of the pristine and optimally doped devices, which is actually a better comparison than the absorption spectrum discussed above. The enhancement in EQE of the galvinoxyl-doped device does not initiate at 430 nm where the galvinoxyl absorption is the strongest. Instead, EQE increases across the entire spectrum. We conjecture that galvinoxyl does not act as a donor molecule in this blend system. 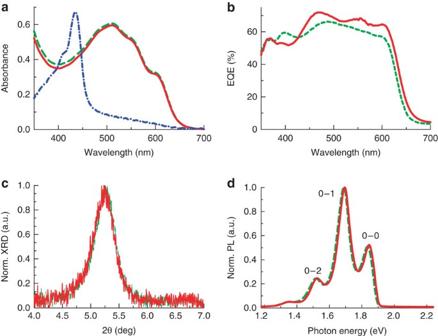Figure 2: Optical and structure properties of pristine and galvinoxyl-doped (3 wt%) P3HT/PCBM blend film and OPV device. (a) The UV/Vis absorption spectrum of pure galvinoxyl (dash–dot line), pristine (dashed line) and doped (solid line) P3HT/PCBM blend. (b) The EQE spectrum of OPV solar cells based on pristine (dashed line) and galvinoxyl-doped (solid line) P3HT/BCBM blend. (c) The XRD pattern of pristine (green dash) and doped (red solid) P3HT/PCBM films. (d) The PL spectrum of pristine (dashed line) and doped (solid line) P3HT/PCBM. The phonon replicas are assigned. Norm., normalized. Figure 2: Optical and structure properties of pristine and galvinoxyl-doped (3 wt%) P3HT/PCBM blend film and OPV device. ( a ) The UV/Vis absorption spectrum of pure galvinoxyl (dash–dot line), pristine (dashed line) and doped (solid line) P3HT/PCBM blend. ( b ) The EQE spectrum of OPV solar cells based on pristine (dashed line) and galvinoxyl-doped (solid line) P3HT/BCBM blend. ( c ) The XRD pattern of pristine (green dash) and doped (red solid) P3HT/PCBM films. ( d ) The PL spectrum of pristine (dashed line) and doped (solid line) P3HT/PCBM. The phonon replicas are assigned. Norm., normalized. Full size image Morphology change and its impact on exciton diffusion towards the D–A interfaces and collection efficiency also have an important role in determining J sc . To investigate whether the film morphology changes due to the addition of galvinoxyl molecules, we compared X-ray diffraction (XRD) patterns of the pristine- and galvinoxyl-doped P3HT/PCBM films ( Fig. 2c ). The XRD (100) P3HT band of both films is the same. Using the XRD peak position, its full width at half maximum, and the Scherrer's relation, we estimate that the average P3HT domain size in both films is ~19 nm. This domain size is ideally suited to the commonly accepted 10 nm exciton diffusion length in the P3HT domains [32] . The relative intensity of 0-0 and 0-1 bands in the photoluminescence (PL) spectrum provides another way to determine the crystallization degree of the P3HT domains [42] . The normalized PL spectra of pristine and doped (3 wt%) P3HT/PCBM films are shown in Fig. 2d . The identical PL spectra indicate that the 'packing order' of polymer chains in the P3HT domains is not affected by the addition of galvinoxyl, and thus the exciton lifetime in the P3HT domains is unchanged. Similar to the XRD and PL results, the transmission electron microscopy (TEM) images ( Supplementary Fig. S1 ) show no observable morphology change caused by the galvinoxyl doping. We therefore conclude that no change in film morphology is responsible for the increase in J sc . To further check the importance of the galvinoxyl spin 1/2 properties rather than its doping ability, we measured OPV device performance with the addition of 'galvinoxyl precursor' molecule that has one extra hydrogen atom, and thus does not possess a spin 1/2 radical (its molecular structure is shown in Supplementary Fig. S2 ). We note that the frontal orbitals are similar in the two molecules, and thus the HOMO–LUMO levels do not change much in going from galvinoxyl to its precursor, as deduced from their similar absorption spectra ( Supplementary Fig. S2 ). In contrast to galvinoxyl doping, we found that doping with this precursor monotonically reduces the OPV device performance ( Fig. 1c ). We therefore conclude that the viable mechanism for the OPV η increase with galvinoxyl additives is suppression of PP recombination at the D–A interfaces due to the spin 1/2 radicals. Galvinoxyl-doped P3HT-rich and PCBM-rich OPV devices To further understand the effect of galvinoxyl doping, we studied OPV cells based on P3HT-rich and PCBM-rich blends. These are P3HT:PCBM at 2:1, 1:2 and 1:5. In P3HT-rich OPV ( Fig. 3a ), η decreases monotonically with doping concentration, indicating that galvinoxyl does not have an enhancement effect on a blend lacking sufficient PCBM acceptor molecules. In contrast, in PCBM-rich system, similar to the standard P3HT/PCBM system, both enhancement and suppression regimes can be clearly identified ( Fig. 3b ). At high galvinoxyl concentration (25 wt%), the doped device performance is still much better than the pristine device. In addition, we notice that the enhancement effect is more significant and the optimal galvinoxyl doping level shifts towards more heavily doping with increased PCBM content. For OPV based on P3HT:PCBM 1:2 blend, η increases by 74% (from 1.08 to 1.88%) at optimal doping of 8 wt%; whereas for devices based on P3HT:PCBM 1:5 blend, η increases by 336% at optimal doping of 15 wt%. In contrast, devices based on pristine PCBM alone did not show any performance enhancement upon galvinoxyl doping. It is thus clear that galvinoxyl enhancement of OPV devices is effective only in the presence of the P3HT/PCBM interfaces. This is consistent with our speculation that galvinoxyl assists the PP dissociation process, which occurs exclusively at the D–A domain interfaces. 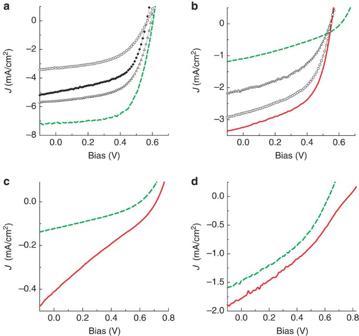Figure 3: I-V characterization of OPV devices based on pristine and galvinoxyl-doped donor/acceptor blends under AM 1.5 illumination. (a) Polymer donor-rich P3HT/PCBM 2:1 blend at various galvinoxyl doping levels: pristine (η=2.8%, dashed line), 1.5 wt% (η=1.9%, triangles), 3 wt% (η=1.6%, diamonds) and 10 wt% (η=1.0%, circles). (b) Fullerene acceptor-rich P3HT/PCBM 1:5 blend at various galvinoxyl doping levels: pristine (η=0.22%, dashed line), 10 wt% (η=0.52%, triangles), 15 wt% (η=0.96%, solid) and 25 wt% (η=0.77%, circles). (c) Regio-random P3HT/PCBM 1.2:1 blend at different galvinoxyl doping levels: pristine (η=0.02%, dashed line) and 3 wt% (η=0.08%, solid). (d) MEH-PPV/PCBM 1:1 blend at different galvinoxyl doping levels: pristine (η=0.26%, dashed line) and 17 wt% (η=0.34%, solid). Figure 3: I-V characterization of OPV devices based on pristine and galvinoxyl-doped donor/acceptor blends under AM 1.5 illumination. ( a ) Polymer donor-rich P3HT/PCBM 2:1 blend at various galvinoxyl doping levels: pristine ( η =2.8%, dashed line), 1.5 wt% ( η =1.9%, triangles), 3 wt% ( η =1.6%, diamonds) and 10 wt% ( η =1.0%, circles). ( b ) Fullerene acceptor-rich P3HT/PCBM 1:5 blend at various galvinoxyl doping levels: pristine ( η =0.22%, dashed line), 10 wt% ( η =0.52%, triangles), 15 wt% ( η =0.96%, solid) and 25 wt% ( η =0.77%, circles). ( c ) Regio-random P3HT/PCBM 1.2:1 blend at different galvinoxyl doping levels: pristine ( η =0.02%, dashed line) and 3 wt% ( η =0.08%, solid). ( d ) MEH-PPV/PCBM 1:1 blend at different galvinoxyl doping levels: pristine ( η =0.26%, dashed line) and 17 wt% ( η =0.34%, solid). Full size image Galvinoxyl-doped OPV devices with other donors and acceptors We carried out additional studies of galvinoxyl doping OPV devices fabricated using blends of other donor and acceptor materials to explore whether the enhancement effect is limited to the P3HT/PCBM system. We replaced the donor polymer in our standard P3HT/PCBM blend with regio-random P3HT (RRa-P3HT), which has a similar chemical structure to regio-regular P3HT except that the hexyl side-chains are arranged randomly. In Fig. 3c, we show that in galvinoxyl-doped (3 wt%) RRa-P3HT/PCBM device, J sc improves from 0.12 to 0.41 mA cm −2 . Coupled with V oc increase from 0.61 to 0.72 V, a 300% increase in η is observed. This is not surprising considering that the dominant loss mechanism in the RRa-P3HT/PCBM blend is PP recombination at the D–A interfaces [43] , a process that galvinoxyl doping is expected to directly suppress [44] . Similar result was obtained when we replaced the donor polymer with poly(2-methoxy-5-(2-ethyl-hexyloxy)-1,4-phenylene-vinylene) (MEH-PPV). In Fig. 3d, we show that J sc of the doped (17 wt%) device increases from 1.47 to 1.78 mA cm −2 . With V oc increasing from 0.63 to 0.78 V, a 30% increase in η is observed in devices based on this blend. In contrast, attempts to enhance η were unsuccessful in OPV devices based on blends with acceptor fullerenes other than PCBM. When we replaced PCBM with bisPCBM, a bisadduct analogue of PCBM or indene-C 60 bisadduct (ICBA) that is a high LUMO level fullerene [9] , we found that η decreases monotonically with galvinoxyl doping. It is worth mentioning that when we replaced a fraction of the PCBM acceptor in the blend with bisPCBM, the enhancement effect was still observable. We thus conclude that PCBM in the organic blend is crucial for effective galvinoxyl doping enhancement. Other radials that we tested but did not show notable enhancement effect in P3HT/PCBM OPV system are: (2,2,6,6-tetramethylpiperidin-1-yl)oxyl (TEMPO), α,γ-bisdiphenylene-β-phenylallyl and bis(1-hydroxy-2,2,4,6,6-pentamethyl-4-piperidinyl) oxalate ( Supplementary Fig. S3, Supplementary Table S2 and Supplementary Methods ). The experimental evidence indicates that the cause for the enhanced η -value in the galvinoxyl-doped OPV devices is the reduced PP recombination rate at the P3HT/PCBM domain interfaces due to the spin 1/2 radical additives. We still need to unravel the mechanism by which galvinoxyl reduces PP recombination. As galvinoxyl is a spin 1/2 radical, we propose a 'spin-flip' mechanism that facilitates PP separation at the P3HT/PCBM interfaces by converting photogenerated PP from spin singlet to triplet ( Fig. 4a ) via spin exchange interaction between the PP and galvinoxyl. As triplet PP has longer lifetime than singlet PP, the enhanced intersystem crossing results in a longer-lived species having a better chance to dissociate. 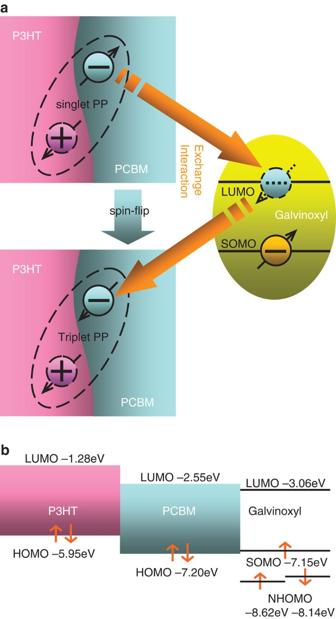Figure 4: Spin-exchange mechanism and DFT calculation. (a) The spin exchange mechanism where the photogenerated PP at the D–A domain interface changes its spin configuration from singlet to triplet augmented by the galvinoxyl spin 1/2 radical. (b) The calculated HOMO, LUMO and SOMO levels of P3HT, PCBM and galvinoxyl that show a clear resonance between the radical and acceptor LUMO levels. Figure 4: Spin-exchange mechanism and DFT calculation. ( a ) The spin exchange mechanism where the photogenerated PP at the D–A domain interface changes its spin configuration from singlet to triplet augmented by the galvinoxyl spin 1/2 radical. ( b ) The calculated HOMO, LUMO and SOMO levels of P3HT, PCBM and galvinoxyl that show a clear resonance between the radical and acceptor LUMO levels. Full size image Consider that a photogenerated exciton in the P3HT domain has spin-up electron in the LUMO level and spin-down hole in the HOMO level. Upon arrival at the D–A interface, the electron transfers to the PCBM LUMO level, forming a singlet PP ( Fig. 4a upper left), with the spin-down hole in the P3HT HOMO level. The singlet PP species can either dissociate into free carriers (polarons) in the P3HT and PCBM separate domains, or geminately recombine. When a spin 1/2 radical such as galvinoxyl, which has spin-polarized singly occupied molecular orbital (SOMO) and LUMO levels with designated spin orientations, is introduced next to the singlet PP, then it may form a complex with PCBM providing a spin-down polarized empty LUMO level in resonance with the spin-up filled PCBM LUMO level next to the charged PCBM molecule ( Fig. 4a right). This mediates an exchange interaction between the up-spin negative polaron and the 'virtual' down-spin of galvinoxyl LUMO that flips the polaron up-spin to down-spin, thereby forming a lower-energy triplet PP ( Fig. 4a bottom left). The PP triplet species has a longer lifetime because it is 'spin-forbidden', having a reduced geminate recombination rate. This may facilitate its dissociation into free polarons. The same mechanism can be equally applied for a photogenerated PP with spin-down electron in the P3HT LUMO level, via exchange interaction with a spin-up defined LUMO level of galvinoxyl radical. We conclude that galvinoxyl additives activate a spin-flip process that converts PP species at the D–A interfaces from spin singlet to triplet, and this reduces the overall PP recombination rate. As our experimental evidence indicates that this process is effective only with the presence of PCBM, and is more effective with increasing PCBM concentration, we therefore believe that galvinoxyl forms a complex with the PCBM at the P3HT/PCBM interfaces. Also the OPV enhancement is maximum at certain galvinoxyl optimal concentration; this can be understood if nearest neighbour galvinoxyl/PCBM complex molecules at high wt% are spin-paired to form spin singlet. Therefore, overdose of galvinoxyl molecules may reduce their ability to provide the spin-flip mechanism necessary for reducing the PP recombination rate. For an effective spin exchange interaction, energy resonance among the charge PCBM and galvinoxyl molecular levels is crucial. To investigate this constraint, we performed density functional theory (DFT) calculations of the ground-state frontier molecular orbital levels of P3HT, PCBM and galvinoxyl using the CAM-B3YP functional. The level alignments among P3HT, galvinoxyl and PCBM are shown in Fig. 4b . P3HT LUMO level (−1.28 eV) is substantially higher than PCBM LUMO level (−2.55 eV), and this facilitates the initial charge transfer that results in PP formation at the D–A interfaces. Importantly, we found that PCBM LUMO (−2.55 eV) is within resonance of the galvinoxyl LUMO (−3.06 eV), and this helps mediating the exchange interaction of the spin-flip process. In addition, the formation of galvinoxyl/PCBM complex may also be important for the spin-flip process. We note that the calculated energy levels are for isolated individual molecules, which may change in forming the complex due to intermolecular interaction. Nevertheless, our calculations show that the energy resonance between galvinoxyl and PCBM is noticeably better than those between TEMPO and PCBM or between galvinoxyl and other acceptors such as bisPCBM and ICBA ( Supplementary Fig. S4 ). This is consistent with our experimental observations that these alternative D–A blends show no significant OPV η enhancement. Finally, we note that spin 1/2 additives may also enhance the electroluminescence (EL) efficiency in organic light emitting diodes (OLED). The ratio of singlet/triplet PP in OLED is usually constrained to be 1:3 due to spin statistics dictated by quantum mechanics. Thus, the number of singlet PPs that are precursors to singlet excitons that ultimately emit EL is severely limited. This is an especially acute problem for OLEDs with blue emission that relies on singlet excitons to yield EL; in particular supplying the missing blue colour for white OLEDs. By adding spin 1/2 radicals to the active layer, we may change the singlet/triplet statistical limit, as the radical may provide another intersystem crossing channel that may increase the singlet PP yield on the expense of triplet PP. This may be a viable route of future investigations, and our results may show the way to advance this research direction because we emphasize the need of energy resonance in the spin exchange mechanism between the spin 1/2 additives and the polaron levels in the active layer. OPV device fabrication The BHJ OPV devices investigated in this study were composed of a transparent indium tin oxide (ITO) anode; a spin-cast polyethylenedioxythiophene/polystyrene sulphonate (PEDOT/PSS) hole transport layer; an active material layer spin-cast from a blend of polymer donor, fullerene acceptor and spin 1/2 radical galvinoxyl (when applicable); and capped with LiF/Al cathode, as shown in Fig. 1a . The ITO-coated glass substrates (Delta Technology, CB-50IN) were cleaned by ultrasonic treatment (in acetone, detergent, deionized water and methanol sequentially) and oxygen plasma treatment. The PEDOT/PSS (Clevios, P VP AI 4083) layer was spin-cast at 5000 r.p.m. for 20 s at ambient conditions and transferred to a nitrogen-filled glovebox (O 2 <1 ppm) for annealing at 120 °C for 30 min. The organic blend that yielded the best device performance ( η ~4%) comprises P3HT (Plextronics, Plexcore OS 2100), PCBM (purity >99.9%) and galvinoxyl (Aldrich, G307). It was prepared in the following way: P3HT (16 mg ml −2 ) and PCBM were dissolved at 1.2:1 weight ratio in 1,2-dichlorobenzene. The blend was heated at 50 °C for 30 min and stirred over night before mixing with galvinoxyl (3 wt%, defined as percentage of total P3HT/PCBM weight) and stirring for 1 additional hour. Other P3HT/PCBM blends were prepared by changing the D–A weight ratio whereas keeping the total P3HT/PCBM mass unchanged. The active layer was spin-cast from the blend at 400 r.p.m. for 6 min and annealed at 150 °C for 30 min. The device fabrication was completed by thermally evaporating a 1-nm thick film of LiF followed by a 100-nm thick film of Al. Each device was 2×2.5 mm in dimension, as shown in Fig. 1a . Finally, the completed device was encapsulated under a cover glass using UV-curable optical adhesive (Norland, NOA 61). Devices using other donor/acceptor materials were fabricated using the same protocol. The PCBM-only device film was spin-cast from a 20-mg ml −1 chlorobenzene solution at 400 r.p.m. and baked at 50 °C for 2 h. The MEH-PPV/PCBM (1:1 weight ratio) film was spin-cast from a 3-mg ml −− toluene solution at 2000 r.p.m. and annealed at 120 °C for 30 min. OPV device characterization Device I-V characteristics were measured using a Keithley 236 Source-Measure unit. The light intensity of the solar simulator, composed of a xenon lamp and an AM1.5G filter, was calibrated at 100 mW cm −2 using a pre-calibrated silicon PV cell. Monochromatic lights used to measure device EQE characteristics were modulated at 36 Hz and filtered by a KG5 filter before sending into the photodetector or OPV device. The photodetector (OPV) device output current was measured using phase-sensitive lock-in technique. MPC measurements When measuring MPC, the OPV devices were transferred to a cryostat that was placed in between the two poles of an electromagnet producing magnetic field, B up to ~200 mT. The devices were illuminated with a tungsten lamp and measured at zero bias using a Keithley 236 apparatus, while sweeping the external magnetic field. The MPC is defined as MPC( B )=[PC( B )/PC(0)−1]. Other characterization methods The absorption spectrum was measured using a UV/Vis spectrophotometer (PerkinElmer Lambda 750) at ambient. XRD was obtained using the Cu K β line and collected by a diffractometer (Philips X'Pert PRO) in powder diffraction mode. PL emission was excited by 100 mW continuous wave laser at 488 nm. The emitted light was collected using a spherical mirror and dispersed by an Acton 300 spectrometer before sending to a photodetector. TEM images were taken under defocused (−25 μm) condition, which is reported to provide enhanced contrast between the P3HT and PCBM regions. Films used for absorbance, XRD and TEM measurements, were prepared in the same way as the active layer of the actual OPV device. Films used for PL measurements were drop-cast from 16 mg ml −1 P3HT solution and annealed at 150 °C for 30 min. DFT calculation The ground state molecular orbital levels were calculated by the Gaussian 09 program [45] with DFT (CAM-B3LYP/6-311g**). The molecular geometry was fully optimized at CAM-B3LYP/6-31g* level [46] , [47] . The DFT calculation for P3HT were performed with periodic boundary conditions [48] (see also Supplementary Methods ). How to cite this article: Zhang, Y. et al . Spin-enhanced organic bulk heterojunction photovoltaic solar cells. Nat. Comm. 3:1043 doi: 10.1038/ncomms2057 (2012).